A strain-absorbing design for tissue–machine interfaces using a tunable adhesive gel To measure electrophysiological signals from the human body, it is essential to establish stable, gentle and nonallergic contacts between the targeted biological tissue and the electrical probes. However, it is difficult to form a stable interface between the two for long periods, especially when the surface of the biological tissue is wet and/or the tissue exhibits motion. Here we resolve this difficulty by designing and fabricating smart, stress-absorbing electronic devices that can adhere to wet and complex tissue surfaces and allow for reliable, long-term measurements of vital signals. We demonstrate a multielectrode array, which can be attached to the surface of a rat heart, resulting in good conformal contact for more than 3 h. Furthermore, we demonstrate arrays of highly sensitive, stretchable strain sensors using a similar design. Ultra-flexible electronics with enhanced adhesion to tissue could enable future applications in chronic in vivo monitoring of biological signals. The ability to precisely measure the electrical signals generated in the living tissue is an important prerequisite for developing medical sensors and diagnostic tools for animate subjects. The signals are usually measured by the direct application of electrodes or probes on biological membranes, almost all of which are inherently soft and exhibit motion. As a consequence, it is difficult to establish good, long-term reliable contact between the device and biotissue by pressing and sticking the devices on biosurface. Further, the hard materials can potentially cause discomfort when placed on the body, as well as induce an inflammatory response when embedded within it. To minimize such negative impacts of hard device materials on biotissue, great efforts have been made to manufacture bioprobes on soft substrates, such as polymers and elastomers. Examples of such soft electronics include two-dimensional multielectrode arrays for sensing electrical signals from the body as well as the pressure, temperature and strain related to it [1] , [2] , [3] , [4] , [5] , [6] . Furthermore, soft sensors that exhibit mechanical flexibility and stretchability can be readily fabricated on three-dimensionally curved surfaces. For example, organic thin-film devices have been manufactured on 1-μm-thick plastic substrates, which exhibit good mechanical robustness, including a minimum bending radius <10 μm (ref. 7 ). Additionally, a flexible active multiplexer for neural probes has been fabricated by thinning silicon and utilizing the transfer printing technology [8] . Finally, a water-soluble adhesive layer based on silk and other adhesive materials has been used to attach ultrathin-film devices directly on the surface of the heart and skin [9] , [10] . By reducing the thickness of stiff materials such as silicon, materials can be made to bend readily; however, this does not change the physical characteristics of the material, such as its Young’s modulus (E). The Young’s moduli of polymeric films are much larger than that of biotissue; The E values of polyimide, collagen and the human brain are ~8 GPa, 100 kPa and 1 kPa, respectively. Therefore, by coating device surfaces with a gel, the initial contact surface can be made softer than polymers or rubber. It also makes the contact surface similar to biotissue. Indeed, single-point probes coated with gel are used widely for recording electromyogram (EMG) and electrocardiogram (ECG) signal from outside the body, as well as the activities of nerve cells within the body. In contrast to the case of body parts that do not exhibit significant movement, such as the brain, signals from those that undergo large movements, such as the heart, are difficult to measure. In particular, the mechanical stress induced in dynamically moving tissue, such as that of the heart, has to be minimized during the measurement. With this goal in mind, Rogers and coworkers have manufactured arrays of multiple sensors, including electric probes, pH sensors and strain sensors on a rubber substrate and have successfully used them to measure heart dynamics [11] . Although electrodes coated with gels are expected to exhibit even better biocompatibility, gels have not been employed during the electrical measurements related to highly deformable parts within the body. This is because none of the currently available biocompatible gel materials exhibit a sufficiently high degree of adhesiveness or mechanical robustness to allow for good mechanical contact between the electrodes and the target organ without causing slippage, delamination or breakage. Here, we report the fabrication of a stress-absorbing active matrix multielectrode array (MEA) on a 1.4-μm-thick polymeric film that can maintain good mechanical contact during electrical measurements under large deformation (over 110% of the compressive strain) of the target object. This is made possible by integrating a photopatternable adhesive gel and organic ultrathin-film-based devices. The gel electrodes are fabricated by dispersing poly(vinyl alcohol) (PVA) in a polyrotaxane matrix. Owing to the extreme flexibility of the substrate and the gel electrode array, the device exhibits conformal contact with a rat heart. The mechanical contact can be sustained for more than 3 h, resulting in a significant improvement in the electronic signal-to-noise ratio. The device can also be removed easily from the heart, when the PVA dissolved in the body. The adhesion strength, duration of contact and conformability of the device can be controlled by varying the molecular weight and degree of saponification of PVA [12] , [13] . Furthermore, the gel electrodes can establish good adhesion on finger joints without necessitating the use of other adhesive materials. This unique characteristic is exploited to measure the bending stress of fingers using a strain sensor coupled with an organic transistor active matrix. This is an important development in the goal of being able to reliably measure vital signals both from within the body and outside it under large deformations. 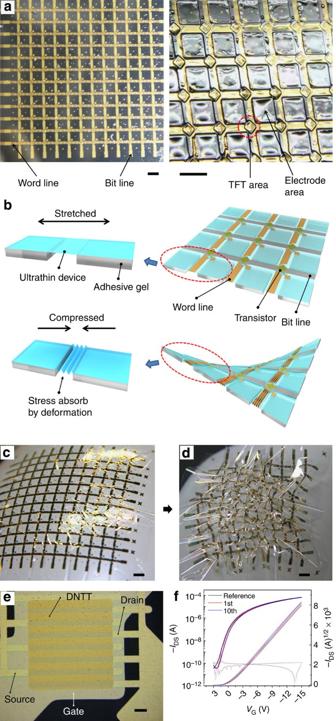Figure 1: Ultrathin OTFT matrix with patterned adhesive gel. (a) Photograph of a 12 × 12 active matrix coupled with adhesive gel electrodes (the entire chip image and the magnified image). The gel covers the transistor and the interconnection pad area in a periodic manner (Scale bar, 5 mm). (b) Schematic illustration of explaining stress-absorbing design using patternable and adhesive gel. (c) Photograph of an active matrix device showing that our design permits stable contact on the surface of a balloon, and under severe compressive strain (100%) (scale bar, 5 mm) (d,e) Microscopy image of a transistor with a top-contact, bottom-gate structure (scale bar, 100 μm). (f) Typical transfer characteristics of the transistor before and after being subjected to 100% compressive strain repeatedly. OTFT, organic thin-film transistor. Design and fabrication Figure 1a shows a schematic of the strain-absorbing, large-area, ultra-flexible MEA, which will be placed directly on the surface of highly deformable biotissue. It also shows a photograph of the entire chip as well as a magnified image of a strain-absorbing MEA with an active matrix of 12 × 12 transistors; the adhesive gel is patterned with precision on the signal-sensing electrodes and the transistor area using ultraviolet radiation. Only the area covered by the photopatterned gel was designed to maintain an adhesive contact during the measurement. During the dynamic and rapid movements of biotissues, such as heart tissue, the induced strain is absorbed by the deformation of the nonadhesive part of the flexible film as well as by the elastic deformation of the part of the tissue that is in contact with the adhesive gel ( Fig. 1b ). Figure 1: Ultrathin OTFT matrix with patterned adhesive gel. ( a ) Photograph of a 12 × 12 active matrix coupled with adhesive gel electrodes (the entire chip image and the magnified image). The gel covers the transistor and the interconnection pad area in a periodic manner (Scale bar, 5 mm). ( b ) Schematic illustration of explaining stress-absorbing design using patternable and adhesive gel. ( c ) Photograph of an active matrix device showing that our design permits stable contact on the surface of a balloon, and under severe compressive strain (100%) (scale bar, 5 mm) ( d , e ) Microscopy image of a transistor with a top-contact, bottom-gate structure (scale bar, 100 μm). ( f ) Typical transfer characteristics of the transistor before and after being subjected to 100% compressive strain repeatedly. OTFT, organic thin-film transistor. Full size image A strain-absorbing MEA was placed on the surface of a balloon ( Fig. 1c ). Even under severe compressive strain (100%), the MEA maintained good mechanical contact (~90% of the pixels remained in contact). Continuous gel films on ultrathin devices are not able to reliably adhere to the surface without selective patterning of adhesive gel due to the lack of strain relief. The compressive strain (100%) was applied for 10 cycles; one of the transistors was characterized, whose magnified image is shown in Fig. 1d after each cycle. The mobility in the saturation regime is 0.67 cm 2 V −1 s −1 at an operating voltage of −15 V. The ON/OFF ratio is 2.3 × 10 5 and the threshold voltage is −1.5 V. The change in the transfer curves ( Fig. 1e ) is negligibly small even after the application of a 100% strain for 10 cycles, demonstrating clearly the strain-absorbing nature of the MEA. The gel pattern formed on the sensing area also helped maintain the ultra-flexible substrate in a relatively flat state, preventing device failure, as the thin gel layer (~40 μm). A biocompatible, photopatternable adhesive gel, referred to hereafter simply as an adhesive gel, was fabricated by dispersing PVA [14] , [15] , [16] , used as an adhesive agent, in a polyrotaxane matrix [17] , [18] , which acted as a UV-cross-linkable gel (see Fig. 2b and Methods). Owing to the increase in the adhesiveness and conformability because of the dispersion of PVA, a sheet of the adhesive gel (area of 8 × 8 cm 2 , thickness of 1 mm, PVA concentration of 5 wt%) could independently support the weight of a coin (5 g) when placed on a hand ( Fig. 2a ); further, the coin did not fall even when shaken vigorously ( Supplementary Movie 1 ). In addition, the adhesive gel could be patterned with UV radiation using a photoinitiator as a cross-linking agent. The patterning of the gel is crucial for realizing multiple isolated electrodes. The patterned gel array could also maintain good contact under severe mechanical deformation (100% compressive strain), as shown in Fig. 1b . Further details are available in Supplementary Fig. 1 . 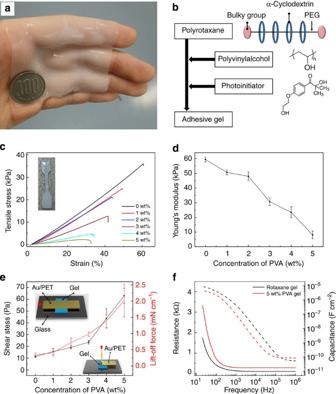Figure 2: Properties of a tunable adhesive gel. (a) Photograph of a large piece of a gel sheet (8 × 8 cm, 1 mm thick) in contact with a hand and supporting a coin (5 g). (b) Adhesive gel, which consists of polyrotaxane, photoinitiator and poly(vinyl alcohol). (c) Typical stress–strain curves of the gels containing different concentrations of PVA, and the shape of the strips used for the measurements (inset). (d) Average Young’s moduli and standard deviation from five samples (error bar) of the gels containing PVA in different concentrations. (e) Average values of the shear stress and peel-off force required to slide (or delaminate) the Au film on the gel and the standard deviation from nine samples (error bar) of values corresponding to nine samples each of the different gels (Inset represents adhesion force measurement setup for lateral direction, top left, and perpendicular direction, bottom right). (f) Resistance and capacitance values of the rotaxane gel and the 5 wt% PVA gel as functions of the frequency, which ranged from 20 to 106Hz (dashed line represents the capacitance). Figure 2: Properties of a tunable adhesive gel. ( a ) Photograph of a large piece of a gel sheet (8 × 8 cm, 1 mm thick) in contact with a hand and supporting a coin (5 g). ( b ) Adhesive gel, which consists of polyrotaxane, photoinitiator and poly(vinyl alcohol). ( c ) Typical stress–strain curves of the gels containing different concentrations of PVA, and the shape of the strips used for the measurements (inset). ( d ) Average Young’s moduli and standard deviation from five samples (error bar) of the gels containing PVA in different concentrations. ( e ) Average values of the shear stress and peel-off force required to slide (or delaminate) the Au film on the gel and the standard deviation from nine samples (error bar) of values corresponding to nine samples each of the different gels (Inset represents adhesion force measurement setup for lateral direction, top left, and perpendicular direction, bottom right). ( f ) Resistance and capacitance values of the rotaxane gel and the 5 wt% PVA gel as functions of the frequency, which ranged from 20 to 10 6 Hz (dashed line represents the capacitance). Full size image Mechanical adhesion and electrical properties of gel To ensure that the device formed a steady contact with biological tissue, we optimized the mechanical and electrical properties of the adhesive gel by varying the concentration of PVA, as discussed later. First, stretching tests were performed to measure the Young’s moduli and maximum tensile stresses corresponding to PVA concentrations ranging from 0 to 5 wt% ( Fig. 2c ). The tensile stress was determined using gel strips (see inset in Fig. 2c and Supplementary Fig. 2c ) and was measured as a function of the strain, which was calculated from the change in strip length. Figure 2d shows the average values of the Young’s modulus and its s.d. for five samples for each PVA concentration. With an increase in the PVA concentration, the Young’s modulus decreases monotonously, reaching 8.4 kPa for the gel with 5 wt% PVA. This value is almost equivalent to the E value of the human brain and only 16% of that of the PVA-free gel (59.4 kPa). The maximum strain, which is defined as the strain at the breaking point, decreases with the increase in the PVA concentration; however, the maximum strain of the gel with 5 wt% PVA (28.2%) was 46% of that of the PVA-free gel (62.3%), as shown in Supplementary Fig. 2d . The unique structure of the rotaxane gel allowed it to be ultrasoft but still stretchable and adhesive [17] , [18] . To quantitatively characterize the adhesiveness of the device shown in Fig. 1 , the lateral and vertical adhesions of the gel to the surfaces of 50-nm-thick Au layers were measured by the tangential shear method [19] , [20] and the 90° peel-off method [21] , respectively. Figure 2e shows the shear stress values as a function of the PVA concentration. With an increase in the PVA concentration from 0 to 5 wt%, the shear stress increases from 11 to 63 Pa. The deviations in the values of nine samples for each concentration were small (10% or less); this was true for concentrations of PVA 3 wt% and lower ( Supplementary Fig. 3a,b ). However, the deviation increased significantly at 4 and 5 wt% PVA, owing to the irregular surface morphology of the resulting gel layers ( Supplementary Fig. 2a,b ). As can be seen in Fig. 2e , the lift-off force, which is defined as the force required to peel off the gel layer, increases from 0.34 to 2.02 mN cm −1 with an increase in the PVA concentration from 0 to 5 wt%. This trend exhibited by the lift-off force is very similar to that shown by the tangential shear values, because the viscosity of a gel is its resistance to deformation by either shear or tensile stress. (See Supplementary Discussion ). The lift-off force data show a fairly wide distribution regardless of the PVA concentration ( Supplementary Fig. 3c,d ). This implies that the adhesion force was not uniform throughout the interface. Figure 2f shows the resistance and capacitance of the various gels; both values depend strongly on the frequency, owing to the low ion mobility in the gels. This trend is also observed in electrical double-layer capacitors [22] , [23] . The increase in the conductivity at higher frequency is similar to what is noticed in ionic gels [24] . The resistance of the 5 wt% PVA gel was higher than that of the PVA-free gel by a factor of two at 5 mV. We believe that polar groups, such as the hydroxyl group of PVA, trap the charged ions in the gel. The resistance of the gel layers increased with a decrease in their thickness [25] . Further details are available in Supplementary Fig. 5 . To investigate the robustness of the adhesive gel under different types of physiological stresses, such as stretching, squeezing and torsion, sheets of the gel with 5 wt% PVA and the PVA-free gel were implanted underneath the skin of a rat. Two sheets of the PVA-free gel were implanted on the right side of the back of a rat parallel to its spine and two sheets of the 5 wt% PVA gel were implanted on the left side ( Fig. 3a ). The rat could move around actively except during magnetic resonance imaging (MRI) observations, which were performed under anaesthesia. 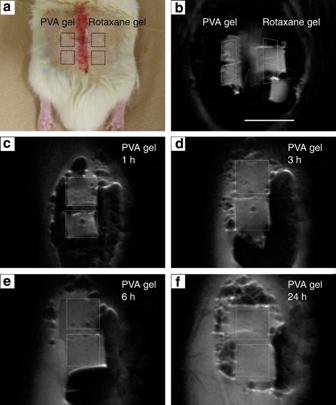Figure 3:In vivoMRI observations of implanted gel pieces. (a) Photograph of a rat showing the positions of the implanted gel pieces. The distance between the pieces of the same gels was 2 mm. (b) MRI image of the pieces of the rotaxane and PVA-containing gels immediately after surgery (scale bar, 2 cm). Images of the PVA-containing gel pieces after (c) 1 h, (d) 3 h, (e) 6 h and (f) 24 h (dashed line represents the original position). Figure 3: In vivo MRI observations of implanted gel pieces. ( a ) Photograph of a rat showing the positions of the implanted gel pieces. The distance between the pieces of the same gels was 2 mm. ( b ) MRI image of the pieces of the rotaxane and PVA-containing gels immediately after surgery (scale bar, 2 cm). Images of the PVA-containing gel pieces after ( c ) 1 h, ( d ) 3 h, ( e ) 6 h and ( f ) 24 h (dashed line represents the original position). Full size image Observation of implanted gel using MRI The positions of the gel sheets were observed using MRI for 1 day. Even during the first MRI observation, which was performed immediately after the implantation surgery, the sheets of the PVA-free gel were found to have moved from their original position ( Fig. 3b ). One hour later, the gel pieces had moved to such an extent that their positions could not be determined using the same scope of MRI system. In sharp contrast, the pieces of the 5% PVA gel did not move at all for 1 h ( Fig. 3c ). After 3 h, the pieces increased in size as they swelled with a liquid and came to touch each other; however, the change in the positions of the two gel pieces was negligibly small ( Fig. 3d ). This result unambiguously shows that the adhesiveness of the PVA-containing gel was maintained for more than 3 h, which is much longer than what we had expected as PVA films normally dissolve within 10 min when placed within the body, owing to the body temperature. The positions of the pieces of the 5% PVA gel moved slightly (the top piece moved left by 2 mm) when the third and the fourth MRI images were obtained after 6 and 24 h, respectively; this was because the adhesive force had decreased ( Fig. 3e,f ). In this way, gels with lower degrees of adhesiveness can be removed easily from the tissue after measurement without causing a large stress or significant damage. Cardiac signal monitoring Next, we attached thin plastic films with MEAs on the surface of the heart of a Wistar rat and performed in vivo cardiac monitoring of the beating heart. A 2 × 2 Au electrode array was fabricated on a 1.4-μm-thick plastic film, and each Au electrode was coated with the 5 wt% PVA adhesive gel. The effective area of the array was 1.5 × 1.5 cm 2 ; these dimensions were comparable to the diameter of the rat heart. For comparison, an array of electrodes not coated with the gel was also prepared. A schematic illustration of the gel-coated MEA, its three-dimensional image, and a microscopic image of the MEA are shown in Supplementary Information ( Supplementary Fig. 6 ). The distance between the electrodes was 1 cm. The heart was surgically exposed via a median sternotomy, and each of the electrodes was contacted on the right and left atria and ventricles. The MEAs exhibited sufficient conformability such that they could be wrapped on the spherical surface of the heart. The average heart rate was ~300 beats per minute during the experiment. The uncoated MEA quickly slipped off the surface of the heart, owing to its repeated and rapid expansion and contraction ( Supplementary Movie 2 ). 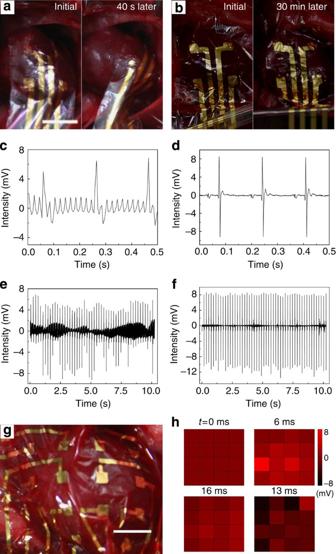Figure 4: Ultra-flexible MEA device and ECG measurement performed using the adhesive gel. (a) Photograph of a conventional device consisting of an array of Au electrodes placed on a rat heart obtained immediately after contact and after 40 s, (scale bar, 1 cm). (b) Photograph of a device consisting of an array of 5 wt% PVA gel-coated Au electrodes placed on a rat heart after contact and 30 min later. Representative voltage signal obtained from the left ventricle for 0.5 s using the Au electrodes (c) and adhesive gel-coated Au electrodes (d), respectively. Representative voltage data from the left ventricle for 10 s using the Au electrodes (e) and PVA gel-coated Au electrodes (f), respectively. (g) Photograph showing that the device (4 × 4 MEA) was in conformal contact with the entire front hemisphere of the rat heart. The distances between the electrodes are 4 mm (lateral) and 3.3 mm (vertical) (scale bar, 4 mm). (h) Simultaneous voltage mapping of a cardiac wave. The signal starts from the right atrium to the outer area. Figure 4a shows images of the uncoated MEA taken immediately after implantation and 40 s after implantation. The MEA moved from the left to the right at an average speed of 2 cm min −1 during 10 repetitions of the test. In contrast, the gel-coated MEA adhered to the heart surface and did not slide even after 30 min ( Supplementary Movie 3 ). Figure 4b shows images of the gel-coated MEA obtained immediately after implantation and after 30 min. The adhesive area always maintained conformal contact with the surface of the heart. Meanwhile, the nonadhesive area underwent repeated folding and unfolding to absorb the stress induced during the cardiac motion. Indeed, many wrinkles were observed, mainly on the nonadhesive area, 30 min after implantation ( Fig. 4b , right). Figure 4: Ultra-flexible MEA device and ECG measurement performed using the adhesive gel. ( a ) Photograph of a conventional device consisting of an array of Au electrodes placed on a rat heart obtained immediately after contact and after 40 s, (scale bar, 1 cm). ( b ) Photograph of a device consisting of an array of 5 wt% PVA gel-coated Au electrodes placed on a rat heart after contact and 30 min later. Representative voltage signal obtained from the left ventricle for 0.5 s using the Au electrodes ( c ) and adhesive gel-coated Au electrodes ( d ), respectively. Representative voltage data from the left ventricle for 10 s using the Au electrodes ( e ) and PVA gel-coated Au electrodes ( f ), respectively. ( g ) Photograph showing that the device (4 × 4 MEA) was in conformal contact with the entire front hemisphere of the rat heart. The distances between the electrodes are 4 mm (lateral) and 3.3 mm (vertical) (scale bar, 4 mm). ( h ) Simultaneous voltage mapping of a cardiac wave. The signal starts from the right atrium to the outer area. Full size image The voltage signal from the heart was measured by combining the gel-coated MEA and a commercial ECG system with an amplifier (MEB-9104, Nihonkohden Co.). The electrical signals from the right ventricle were measured using the uncoated and gel-coated MEAs, as shown in Fig. 4c,d , respectively. In the case of the uncoated MEA, the maximum signal amplitude fluctuated between 5 to 7 mV, with the noise level being ~1.5 mV. In contrast, the maximum amplitude in the case of the PVA-coated MEA was almost constant (8 mV), with the noise level being 0.1 mV. The signal measured with the gel-coated MEA ( Fig. 4d ) exhibits all of the P, Q, R, S, T and U waves. In the case of uncoated MEA ( Fig. 4c ), the noise spoiled the P, T and U waves, though the T wave is essential in the diagnoses of cardiac ischaemia and infarction. The voltage signals were monitored for a longer period to determine the reliability of the measurements. For the uncoated MEA, 51 peaks were counted over 10 s; the average maximum amplitude was 4.7 mV and the s.d. was 0.85 mV ( Fig. 4e ). In contrast, for the gel-coated MEA, 53 peaks were recorded over the same period; the average maximum amplitude was 8.1 mV and the s.d. was 0.28 mV ( Fig. 4f ). Thus, the use of the gel-coated MEA resulted in improved signal intensity, reliability and sensitivity as reliable contacts could be formed and maintained throughout the experiment. In addition, we measured ECG using platinum (Pt) MEA to check the electrode material dependence. However, signal quality and sliding behaviour was almost the same as the Au MEA ( Supplementary Fig. 7 ). We think the electrode material does not have a strong influence on the signal quality when the contact is not stable. Structural modification, such as open mesh layout could be a good alternative method to improve stable contact on biological tissue. We performed the same experiment on four rats to establish the reproducibility. All the devices without PVA gel coating showed sliding behaviour and lower signal quality. The cardiac signal was mapped in real time using a 4 × 4 gel-coated MEA, which covered a hemispherical surface ( Fig. 4g ). In this experiment, the fabricated MEA was removed from the supporting substrate and immediately attached to the surface of the heart to prevent the adsorption of contaminants ( Supplementary Fig. 8 ). The temporally varying cardiac signal was mapped for several cycles (see Fig. 4h and Supplementary Movie 4 ). A rat’s heart beats five times per second, with the volume of the heart changing by ~30%. Further, the bending radius of the heart is ~8 mm, and the surface of the heart is very slippery. Given these facts, it is not possible to form and maintain good contacts with the heart and obtain reliable data without using an adhesive gel. Surface potential mapping using the gel-coated MEA will provide a valuable evidence for identifying the site of origin of arrhythmias, especially in the case of re-entry arrhythmia. The device will also be applicable to mapping of conduction in a heart with malformation. When an examination using conventional catheter electrodes does not draw definitive information for such abnormalities, the surface potential mapping is expected to provide an additional diagnostic modality. Maintaining the conformal contact of the electrodes is crucial for an accurate diagnosis. Application on human skin In addition to being useful in in vivo applications, adhesive gels can be used to form reliable contact between electronic devices and human skin. To detect the strain induced by the motion of the body, highly sensitive, stretchable strain sensors were fabricated. The printable elastic conductor used [26] comprised fluorinated copolymer, Ag flakes, graphene and an ionic liquid dispersed in 4-methly-2-pentanone. The paste formed from these components was highly viscous and was patterned on a polydimethylsiloxane (PDMS) substrate by the blade coating method ( Fig. 5a and Methods). 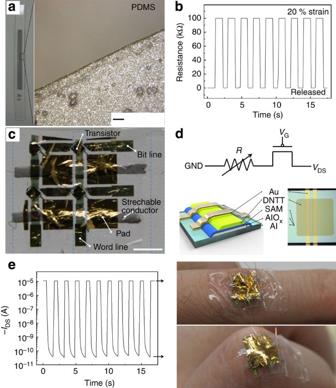Figure 5: Stretchable motion sensor integrated with an organic transistor. (a) Photograph of a stretchable conductor printed on a PDMS substrate and optical microscopy image of their interface (scale bar, 100 μm). (b) Resistance of the printed conductor as it is subjected to repeated stretching (20%) and relaxation. (c) Image of a 2 × 2 array of strain sensors on a PDMS substrate. (The blue line represents the PVA gel, scale bar, 5 mm) (d) Circuit diagram of the motion sensor and schematic illustration and optical microscopy image of an organic transistor. (e) ON current behaviour of the transistor under repeated folding and unfolding of the finger. Figure 5: Stretchable motion sensor integrated with an organic transistor. ( a ) Photograph of a stretchable conductor printed on a PDMS substrate and optical microscopy image of their interface (scale bar, 100 μm). ( b ) Resistance of the printed conductor as it is subjected to repeated stretching (20%) and relaxation. ( c ) Image of a 2 × 2 array of strain sensors on a PDMS substrate. (The blue line represents the PVA gel, scale bar, 5 mm) ( d ) Circuit diagram of the motion sensor and schematic illustration and optical microscopy image of an organic transistor. ( e ) ON current behaviour of the transistor under repeated folding and unfolding of the finger. Full size image The conductivity of the paste was measured using the four-probe method and found to be 10 4 S cm −1 . This paste was printed on a PDMS substrate and covered with another piece of PDMS to form resistors (length: 1 cm, width: 1 mm, thickness: 10 μm) sandwiched between two PDMS sheets. The resistance of these resistors was measured while they were repeatedly stretched and released ( Fig. 5b ). The resistance was 20 Ω at a strain of 0% and increased linearly with the strain till up to 10%. However, when the strain exceeded 15%, the resistance increased exponentially and reached the maximum measurable value at a strain of 20% ( Supplementary Fig. 9a ). Small cracks were observed for strains >10%, and the number of cracks increased significantly for strains >15%. A few parts of the printed conductor came to be disconnected owing to the cracks ( Supplementary Fig. 10 ). However, it is worth noting that the resistance returned to the original value once the stress was released. A cyclic test involving subjecting the resistors to a 20% strain and then releasing the strain was performed more than 1,000 times. The measured resistance values exhibited good reproducibility, with the relative change in the resistance being of the order of 10 4 and greater. For a motion sensor demonstration, we integrated a 2 × 2 active matrix of transistors with an array of strain-sensor pixels ( Fig. 5c ). The pixels were printed using a stretchable conductor whose resistance changes with the strain and were fabricated on 2-μm-thick PDMS films. They were pre-stretched by ~25% and then integrated with the active matrix. The circuit diagram of the motion sensor and the architecture of the organic transistor are shown in Fig. 5d . The typical transfer characteristics of the transistors are shown in Supplementary Fig. 9c . The mobility in the saturation regime was 1.5 cm 2 V −1 s −1 , the ON/OFF ratio was 7 × 10 5 and the threshold voltage was −0.37 V at the operation voltage of −2 V. The output characteristics of the transistors are shown in Supplementary Fig. 9b . This device was gently attached to the joint of a finger for measurement after the completion of the gel-patterning process. A schematic illustration of the device structure is shown in Supplementary Fig. 9d . The PVA gel was patterned under the PDMS sheet, which was subjected to a plasma treatment to enhance the adhesion of the gel on the device. The device was then continuously stretched (~20%) and released by the folding and unfolding motion of the finger. The presence of the thin layer of the PVA gel enabled soft and conformal contact on the skin and prevented the device from sliding during the repeated movements. We measured the ON current of the transistor under a constant drain and gate voltages of −2 V. The change in the resistance of the stretchable conductor, which was connected between the ground and the source of the transistor, switched the transistor on, generating the ON current, as shown in Fig. 5e . The ON current exhibited a difference of an order of 10 5 in magnitude during the different stages of the repeated motion of the finger. We discussed the possibility of controlling the adhesion force and lift-time of the adhesive gel under various conditions during the in vivo experiment by modifying the gelation method used. Indeed, the mechanical properties and morphology of the adhesive gel could be controlled by varying the concentration of PVA in the gel. The highest mixing gel/PVA ratio (w/w) used was 2:1; however, this resulted in a very high degree of interference in gel cross-linking. As the PVA concentration was increased, the roughness of the gel and the frictional force both increased ( Supplementary Fig. 2a,b ), resulting in an increase in the adhesive force [27] , [28] . The adhesive force of the gel increased exponentially with the PVA concentration. Further, the gel exhibited good uniformity and a stretchability of ~30% ( Supplementary Fig. 2d ). We attribute this to the unique stress-equalizing ability of the rotaxane gel [17] , [18] , because the cross-links formed pass along the polymer chain like a pulley, allowing any stress formed to be uniformly distributed through the many cross-linking points. We also attempted to determine why the gel did not separate from the target parts in a moving rat even after several hours, as was determined from the MRI scans; this duration was much longer than the typical dissolving time (10 min) of PVA at body temperature. To understand the reason for this, the lateral adhesive force between the gel and a biotissue (pig muscle tissue) was measured by the tangential shear method and compared with that between the gel and Au surface ( Supplementary Fig. 3 ). In spite of the gel/biotissue interface being wet, the adhesive force at the interface was five to six times higher than that at the gel/Au interface. This can be ascribed to the fact that the rough surface of the biotissue improved adhesion. Further details are available in Supplementary Information ( Supplementary Fig. 4 ). More importantly, both the biotissue and the gel exhibited elastic deformation (~2 mm displacement) before the gel/biotissue interface started to slide and come apart. This resulted in the shear stress curve reaching a plateau slowly ( Supplementary Fig. 4a ), unlike the curve for the gel/Au interface. Although the implanted device will always be subjected to stress resulting from the movement of the tissue, it should be able to accommodate small stresses owing to the elastic deformation of the soft gel and the tissue, with the gel/biotissue interface remaining intact. In this way, a small adhesive force could result in good contact for a long period, as confirmed by the MRI observations. Preparation of adhesive gel solution and patterning Modified polyrotaxane (1 g) (AOI-E2-APR100, Advanced Softmaterials Inc.) was suspended in distilled water (10 ml, 40 °C) and stirred until it had dissolved completely. Next, the photoinitiator (0.2 g) 4-(2-hydroxyethoxy)phenyl-(2-hydroxy-2-propyl)ketone (Irgacure 2959, Ciba Specialty chemicals Inc.) was added to the solution under constant stirring to obtain a homogeneous mixture. Finally, PVA (0.1, 0.2, 0.3, 0.4 or 0.5 g) (Kuraray, M w : 87,000–127,000; degree of saponification: 87–89%) was added to the solution, and the solution was stirred for 10 h to ensure it was homogeneous. Prepared solution was casted on the device, which is oxygen plasma treated (300 W, 30 s) and covered by glass. The gel thickness was controlled by spacers between the device and glass, and patterning was performed by using a metal mask to cover the glass. Finally, the solution was cross-linked by ultraviolet irradiation (Optical Modulex, Ushio) with 250 W and 365 nm for 1 min. Measurement of mechanical properties The test gel strips were prepared using a PDMS mould with a thickness of 2 mm and a width of 1.5 mm in its middle (see inset of Fig. 2c ). The Young’s moduli of the gel strips were measured using a dynamic mechanical analyser from Shimadzu (Ag-X). The gel strips were stretched at a constant rate of 4 mm min −1 . Measurement of adhesive properties A PDMS layer (1 mm) was used as a supporting layer for a 1.4-μm-thick polyethylene terephthalate (PET) foil (Mylar 1.4 CW02, Pütz GMBH+Co.). Next, a thin film of Au (20 nm) was deposited on the PET film. The PET film was then placed in conformal contact with the gel strip, which was fixed on a glass substrate; the contact area was 1 cm 2 . Then, the film was pulled using a dynamic mechanical analyser instrument at a constant rate of 4 mm min −1 to measure the tangential shear stress ( Supplementary Fig. 3a ). A piece of commercial pork shoulder muscle was fixed on a glass substrate using double-sided adhesive tape. The gel patterned on the PET film was placed in conformal contact with the pig tissue; the contact area was 1 cm 2 . The film was then pulled at the same rate, that is, at 4 mm min −1 . The surface of the pig tissue was kept sufficiently wet during the measurement to prevent it from drying. In the case of the 90° peel-off measurements, the prepared Au film was placed in contact with a gel strip bent at an angle of 90°. The supporting PDMS layer at the contact area was removed to minimize the residual stress from bending. Then, the Au film was laminated in the same manner ( Supplementary Fig. 3c ). Impedance measurement The impedances of the rotaxane and PVA gels were measured using metal–insulator–metal structures and an I – V parameter analyser (Agilent, 4156C) as functions of the frequency (20 to 10 6 Hz). A 1-mm-thick ion–gel layer was sandwiched between an Au-deposited polyimide substrate; the top-contact area was 1 cm 2 . The measurements were repeated for alternating current voltages of 5–1,000 mV. Fabrication of passive electrode An array of Au electrodes and interconnect lines were deposited on a PDMS-supported 1.4-μm-thick PET foil using a thermal evaporator. A thin layer (1 μm) of parylene (diX-SR, Daisankasei) was then deposited on the structure by chemical vapour deposition (CVD) to isolate the entire structure except the electrode area. For the UV patterning of the gel, the gel solution was poured on the substrate. A glass slide was used to spread the solution at a distance of ~70 μm from the substrate using a tape spacer. The electrode area was exposed to ultraviolet radiation for 1 min using a shadow mask. The remaining solution on the unexposed area was removed by dipping the substrate in water. The electrodes were connected to an amplifier (MEB-9104, Nihonkohden Co.) to monitor the ECG signal from the rat heart. Animal experiments The research protocol for the use of rats followed the University of Tokyo’s Regulations for Animal Care and Use, which were approved by the Animal Experiment Committee of the Institute of Medical Science, the University of Tokyo. We used 10-week-old rats. The rats were placed under general anaesthesia using isoflurane; an anaesthesia tube was placed into the trachea. During the surgical procedures, we used commonly accepted intraoperative management techniques. The body temperature was maintained at 37 °C using a heating pad. To approach the surface of the heart, we opened the chest with a median incision. The breastbone was kept apart using a rib spreader. MRI studies MRI scans were obtained using the Turbo-RARE method. A 7-T MRI system (BioSpec 70/20 USR, Bruker Co.) was employed for the purpose. To ensure that the PVA gel strips were noticeable in the MRIs scans, the acquisition parameters were adjusted to the following T2-weighted levels: repetition time ( T R ) of 2,500 ms and an echo time ( T E ) of 33 ms. The original positions of the gel strips were marked on the skin. Motion sensor and active matrix fabrication Ag flakes (2 g, Sigma Aldrich); a fluorinated copolymer, vinylidene fluoride-tetrafluoroethylene-hexafluoropropylene, (0.5 g, Daikin Industries, Daiel-G912); an ionic liquid, 1-ethyl-3-methylimidazolium tetrafluoroborate (0.05 g); and graphene ink (prepared by Jokoh, Japan) (0.2 g, dispersed in a 4-methyl-2-pentanone in an amount of 10 wt% by jet milling at 10 MPa over 10 passes) were mixed over 16 h in 4-methyl-2-pentanone (1.5 g). The resulting paste-like ink was then printed on a thin PDMS substrate with a thickness and width of ~10 and 1,500 μm, respectively. Then, a 2-μm-thick layer of PDMS was coated all over the ink pattern except for the area where the transistor matrix and the wire were connected. The bottom side of the PDMS layer was treated with an oxygen plasma (300 W, 30 s) and a layer of the PVA gel (10 mm × 1 mm, thickness of ~30 μm) was patterned on it. The active matrix of organic transistors was fabricated on a 1.4-μm-thick PET film supported by a polymer layer. First, a 20-nm-thick Au layer was thermally deposited as a word line on the substrate. Then, a 200-nm-thick parylene layer was formed by CVD. Next, a 30-nm-thick DNTT (dinaphtho[2,3-b:2',3'-f]thieno[3,2-b]thiophene) organic active layer was deposited by evaporation using a shadow mask. After that, a 50-nm-thick Au layer was deposited using a shadow mask to form the source and drain and the interconnection. Parylene was deposited through CVD for encapsulation. A via hole was drilled in it using a laser. Finally, Au was thermally deposited on the pad to connect it with the gel electrodes. The active matrix for the low-voltage motion sensor had a different structure. First, a 20-nm-thick aluminium (Al) layer was evaporated as a word line on a 1.4-μm-thick PET film. Then, a 4-nm-thick aluminium oxide (AlO x ) layer was formed on the Al layer by treating it with oxygen plasma (300 W, 5 min). The AlO x layer was covered with a 2-nm-thick self-assembled monolayer (SAM) by dipping the substrate into a solution of 2-propanol containing 5 mM n-tetradecylphosphonic acid for 16 h at room temperature. This gate dielectric has a large capacitance (700 nF cm −2 ) and exhibits small leakage currents. Following processes after gate insulator are the same with above active matrix fabrication method. A printed conductor was integrated with the matrix while being pre-stretched by 25%. All the electrical measurements were performed in air using a semiconductor parameter analyser (4156C, Agilent). How to cite this article: Lee, S. et al. A strain-absorbing design for tissue–machine interfaces using a tunable adhesive gel. Nat. Commun. 5:5898 doi: 10.1038/ncomms6898 (2014).